A fully atomistic computer simulation study of cold denaturation of a β-hairpin Cold denaturation is a fundamental phenomenon in aqueous solutions where the native structure of proteins disrupts on cooling. Understanding this process in molecular details can provide a new insight into the detailed natures of hydrophobic forces governing the stability of proteins in water. We show that the cold-denaturation-like phenomenon can be directly observed at low temperatures using a fully atomistic molecular dynamics simulation method. Using a highly optimized protein force field in conjunction with three different explicit water models, a replica exchange molecular dynamics simulation scheme at constant pressures allows for the computation of the melting profile of an experimentally well-characterized β-hairpin peptide. For all three water models tested, the simulated melting profiles are indicative of possible cold denaturation. From the analysis of simulation ensembles, we find that the most probable cold-denatured structure is structurally compact, with its hydrogen bonds and native hydrophobic packing substantially disrupted. Cold denaturation of proteins is an intriguing property of globular proteins that lose their native structures on decreasing temperature. Unlike heat denaturation, whereby a native protein is disrupted at high temperature, cold denaturation is accompanied by decreases in both the system entropy and enthalpy. One possible explanation for this thermodynamic behaviour is a substantial ordering of water molecules around exposed hydrophobic residues and subsequent enhancement of the hydrogen bond network of shell water [1] , [2] . As the weakening hydrophobic force with decreasing temperature appears to be a key driving force governing cold denaturation, investigations of cold denaturation using either experimental or computational methods can provide new insights into the nature of hydrophobic effects. The thermodynamics of cold denaturation has been well-characterized experimentally for several globular proteins by calorimetric [3] , circular dichroism [4] , [5] , and nuclear magnetic resonance (NMR) [6] , [7] experiments. Notably, the cold-denatured structure of ubiquitin was fully determined using a pressure-assisted NMR method [8] . In the area of computational biophysics, all-atom-level molecular dynamics (MD) simulation has been shown to be a viable computational tool, as it can provide detailed atomistic pictures of complex molecular systems and allow direct comparisons with thermodynamic/kinetic experimental data. Despite growing computational power and recent advances in simulation methods, all-atom MD studies directly targeting cold denaturation are rare. In fact, only a few computer simulations have been performed on this topic [2] , [7] , [9] . In earlier studies, a simple coarse-grained MD on a two-dimensional homopolymer model was applied in an effort to probe the microscopic origin of cold denaturation [2] . Also, an enhanced MD incorporating generalized Born (GB) implicit solvation was employed to simulate the cold denaturation of a series of β-hairpin peptide models [7] . However, care should be taken when interpreting such results based on the implicit water model, because in principle this model cannot properly take into account the combined effect of enthalpy and entropy changes associated with temperature variations [1] and hence simulation results obtained from the implicit solvation model can be misleading. In this regard, explicit treatments of water appear to be essential to elucidate the role of water governing hydrophobic interactions of proteins. Most recently, using an explicit water model in a coarse-grained level, a three-dimensional lattice simulation of hydrated proteins was performed to simulate cold and heat denaturation [9] . Although an all-atom MD scheme with explicit treatment of water solvation offers a better computational strategy for cold denaturation, previous all-atom simulations have been limited to probing cold-denaturation states indirectly based on extrapolations of simulation data to low temperatures [10] , [11] . Until now, however, direct observations of cold denaturation using all-atom MD have not yet been reported. In this work, we attempt to demonstrate in silico cold denaturation using a fully atomistic MD approach. For a comprehensive demonstration of the cold-denaturation phenomenon, a β-hairpin forming peptide (MrH1) is chosen as a benchmark model system. This model peptide contains a total of 16 residues, of which 6 are hydrophobic (TYR3, VAL5, ILE7, ILE12, VAL14 and ILE16). Furthermore, a single hydrophobic cluster formed by these non-polar residues provides the major stabilizing factor of the β-hairpin structure in water [12] . Under ambient conditions, MrH1 is marginally stable in water (a folding fraction of about 50%), but when the temperature is decreased from the temperature of maximum folding fraction ( T max =303 K), this peptide displays a gradual loss of the native structure, as shown by its NMR-based melting profile (folding fraction versus temperature) [12] . On the basis of the thermodynamic ground of protein stability, characteristic features of cold denaturation can be investigated by producing these melting curves. To simulate melting profiles, relevant protein conformations need to be fully explored over an extended temperature range, including below 0 °C. For this purpose, an accelerated MD scheme effectively operating in a broad range of temperature is warranted. Herein, we apply a state-of-the-art replica exchange molecular dynamics (REMD) simulation using the isothermal–isobaric ensemble (NPT ensemble). The constant pressure REMD is chosen primarily to incorporate natural changes in system density caused by variations in temperature. As for the force field, we use the ff99sb-nmr1-ildn force field (nmr1) [13] , [14] for the protein segment. The nmr1 force field is a highly optimized version of its parent force field ff99sb [13] and is obtained by best fit to the NMR chemical shift data of several test proteins. Here, a side-chain torsional correction term independently optimized by Shaw et al. (ildn) [14] is added. As for the explicit water model, three different water models, namely, tip3p (ref. 15 ), tip4p/2005 (ref. 16 ), and tip4p/ ε (ref. 17 ), are employed. The tip3p model has been widely used for biomolecular simulations, but its temperature-dependent properties such as density, isothermal compressibility and heat capacity deviate significantly from experimental values [18] , [19] . In contrast with the tip3p model, the tip4p/2005 model [16] (an improved version of its parent tip4p model [15] ) can reproduce various experimental temperature-dependent properties. Especially, this model gives an excellent water density profile over the temperature range −20≤ T ≤100 °C. However, a major defect of tip4p/2005 is an underestimation of dielectric constant of water ( ε =58 at 298 K). The tip4p/ ε model is another modified version of the tip4p model and its performance is nearly comparable to that of tip4p/2005, but notably for tip4p/ ε , the dielectric constant of water was refined to match experimental values over an extended temperature range. From this simulation protocol stated above, we successfully reproduce qualitatively correct pictures of cold denaturation and identify possible cold-denatured structures at low temperatures. The current study is of importance in that the scope of all-atom MD simulations has been expanded into proteins at cold temperatures. Also, in conjunction with recent experimental progress in determination of three-dimensional cold-denatured structures of globular proteins [8] , this simulation protocol can open the door for optimizing all-atom force fields against cold-denatured structures of such proteins beyond their native structure. 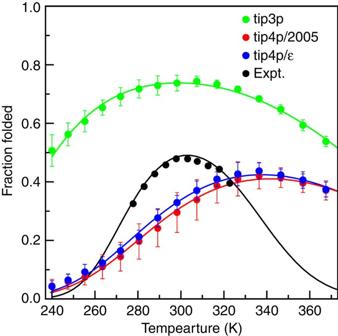Figure 1: Simulated melting curves in comparison with the NMR experiment. The green, red and blue open circles denote the results obtained using tip3p, tip4p/2005 and tip4p/ε, respectively. The temperature of maximum folding fraction (Tmax) is 307 K for tip3p, 340 K for tip4p/2005 and 336 K for tip4p/ε. The black filled circle shows the NMR-based result.12The solid lines are the results from a two-state model fit. The error bar is estimated at the 95% confidence level. Melting curves indicative of cold denaturation Figure 1 shows the simulated melting curves of MrH1 (−33≤ T ≤100 °C) using the three explicit water models. In this temperature range, all three water models represent a liquid state. As expected from the typical parabolic feature with maximum folding fraction at T max , the folding fraction obtained from each water model consistently decreases as the temperature is lowered below T max . This observation indicates that all these water models produce cold denaturation. In particular, it is notable that the tip3p model leads to cold denaturation despite its poor temperature dependence [18] . Compared with the tip3p model, both tip4p/2005 and tip4p/ ε yielded melting curves that are closer to the experimental values, probably owing to their better treatments of temperature dependence. Thus, for the simulation of cold denaturation, accurate modelling of the temperature dependence of water is probably an important factor for consideration, but not a necessary one. Figure 1: Simulated melting curves in comparison with the NMR experiment. The green, red and blue open circles denote the results obtained using tip3p, tip4p/2005 and tip4p/ ε , respectively. The temperature of maximum folding fraction ( T max ) is 307 K for tip3p, 340 K for tip4p/2005 and 336 K for tip4p/ ε . The black filled circle shows the NMR-based result. [12] The solid lines are the results from a two-state model fit. The error bar is estimated at the 95% confidence level. Full size image From the simulated melting curves, thermodynamic parameters were obtained by best fit to a two-state folding model [12] ( Table 1 ). Consistent with the NMR-based result, the predicted and on unfolding are both negative. The positive heat capacity change Δ C ° p is indicative of a possible disruption of the hydrophobic cluster on unfolding; the underestimation of Δ C ° p results from the flattening of calculated melting curves ( Fig. 1 ). Although there is a quantitative gap between theory and experiment, all simulated thermodynamic quantities reproduce qualitatively correct thermodynamic features of cold denaturation. Table 1 Thermodynamic parameters on unfolding. Full size table Direct comparisons with the experimental melting profile [12] showed that all simulated melting curves were consistently broadened. Furthermore, the tip3p model showed the up shift, whereas both tip4p/2005 and tip4p/models showed the right shift. Interestingly, these deviation patterns are similar to the well-known stability feature of thermophilic versus mesophilic proteins [20] . In this regard, we anticipate that intrinsic force field biases in the present simulation appear to enhance thermal stability of the MrH1 peptide. One possible source of such biases is the overestimation of hydrophobic interactions by the current force field. This view is in line with prior simulation results that showed that the hydration free energies of non-polar molecules are systematically overestimated [19] , [21] , [22] , [23] . In an effort to remedy such discrepancies, relevant protein/water interaction terms in the force field may need to be further optimized. Transition from the native to possible cold-denatured state Having demonstrated the possibility of simulating the cold-denaturation-like phenomenon with the present simulation protocol, we investigated conformational transitions from the native to possible cold-denatured states during the cooling process. For that purpose, a conformational probability distribution for each water model ( Fig. 2 ) is given as a function of the protein backbone root mean square deviation (RMSD) from the NMR model ( Supplementary Fig. 1 ). In the case of the tip3p model ( Fig. 2a ), the native state (RMSD=1.0 Å) at T max is most populated. On cooling from T max (307 K) to T low (240 K), the native population decreases, but the population of the non-native state near RMSD=2.1 Å increases. Most likely, this particular non-native state could be located as a dominant cold-denatured state if the temperature further decreases below T low . In the case of modified tip4p models, much clearer pictures of cold-denatured states can be obtained. As illustrated in Fig. 2b (tip4p/2005) and Fig. 2c (tip4p/ ε ), when the temperature decreases from T max to T low , the major population gradually shifts from the native state (RMSD=1.0 Å) to the non-native state (RMSD=2.5 Å). This transition to the non-native state is a common feature for both modified tip4p models. 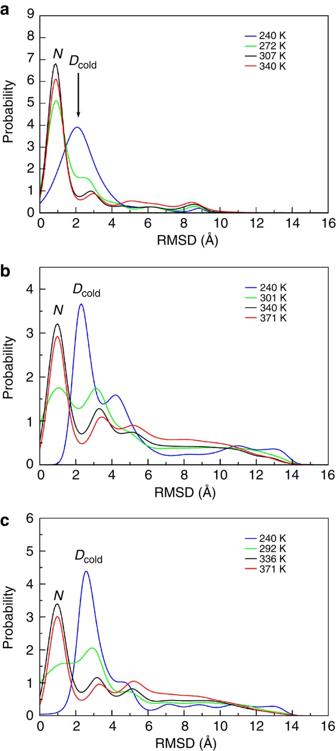Figure 2: Probability distribution in RMSD space on cooling. The conformational probability distributions of the peptide were shown as a function of the backbone RMSD from the NMR native model. Four different temperatures were considered. The symbols ‘N’ and ‘Dcold’ denote the native and possible cold-denatured states, respectively. These distribution functions were computed for three explicit water models: (a) tip3p. (b) tip4p/2005. (c) tip4p/ε. Figure 2: Probability distribution in RMSD space on cooling. The conformational probability distributions of the peptide were shown as a function of the backbone RMSD from the NMR native model. Four different temperatures were considered. The symbols ‘ N ’ and ‘ D cold ’ denote the native and possible cold-denatured states, respectively. These distribution functions were computed for three explicit water models: ( a ) tip3p. ( b ) tip4p/2005. ( c ) tip4p/ ε . 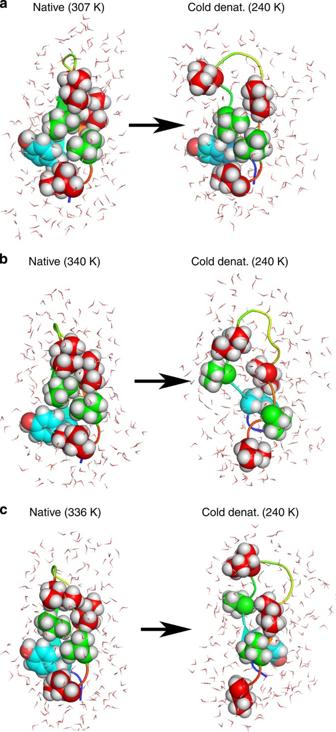Figure 3: The major conformational change on cooling. From cluster analysis24of the simulation ensemble at ambient and low temperatures, the centre structure of the most populated cluster was selected as representative at each temperature. In those major conformational clusters at low temperatures, the native type I’ turn of MrH1 changed to a bulged loop as the hydrophobic cluster is disrupted. For definition of distinctive clusters, an RMSD criterion of 2.5 Å was used. The six hydrophobic residues were drawn using a space-filling model (red, ILE; green, VAL; Cyan, TYR) and a stick model was used to represent surrounding water molecules. Three explicit water models are used: (a) the tip3p model (Tmax=307 K andTlow=240 K). (b) the tip4p/2005 model (Tmax=340 K andTlow=240 K). (c) the tip4p/εmodel (Tmax=336 K andTlow=240 K). Full size image Characterization of possible cold-denatured structures Figure 3 shows the representative conformation of the cold-denatured-like state for three water models and the native structure. Hierarchical cluster analysis [24] was applied to find distinctive conformational clusters from the simulation ensembles taken at two different temperatures ( T max and T low ). This cluster analysis showed that native-like structure (RMSD=1.0 Å) belongs to the most populated cluster at T max . However, as the temperature was decreased from T max to T low , a non-native structure (RMSD=2.1 Å for the tip3p model or 2.5 Å for the tip4p models) was at the centre of the major conformational cluster and was therefore defined as one possible representative of the cold-denatured state. For minor conformational clusters of the cold-denatured state, the structural integrity of the β-strand is more disturbed (See Supplementary Fig. 2 for more details). As shown in Fig. 3 , the native hydrophobic cluster is composed of six non-polar residues and is tightly packed. For the tip3p model, its cold-denatured-like state at T low exhibits disruption of only the hydrophobic interaction pair of ILE7 and ILE12 near the turn region. For both tip4p/2005 and tip4p/ ε , however, the cold-denatured-like state gives rise to more disruption of the hydrophobic cluster with a substantial loss of the native hydrogen bonds, but remains to be structurally compact. This finding is consistent with a previous NMR result of a mutant of MrH1 in a mixture of hexafluoro-2-propanol/water [25] . Figure 3: The major conformational change on cooling. From cluster analysis [24] of the simulation ensemble at ambient and low temperatures, the centre structure of the most populated cluster was selected as representative at each temperature. In those major conformational clusters at low temperatures, the native type I’ turn of MrH1 changed to a bulged loop as the hydrophobic cluster is disrupted. For definition of distinctive clusters, an RMSD criterion of 2.5 Å was used. The six hydrophobic residues were drawn using a space-filling model (red, ILE; green, VAL; Cyan, TYR) and a stick model was used to represent surrounding water molecules. Three explicit water models are used: ( a ) the tip3p model ( T max =307 K and T low =240 K). ( b ) the tip4p/2005 model ( T max =340 K and T low =240 K). ( c ) the tip4p/ ε model ( T max =336 K and T low =240 K). Full size image Snapshots of free-energy landscape on cooling Investigations of free-energy landscapes during cold denaturation are of interest, because tracing topographical changes of the free-energy surface on cooling can provide clear views on the cold-denaturation-like phenomenon. As proper reaction coordinates for free-energy representations, we employed the number of the native backbone hydrogen bond ( N HB ) and the solvent accessible surface area of the non-polar component (SASA_np) [26] . The free-energy surfaces at several temperatures obtained from tip4p/2005 are given as functions of (RMSD, N HB ) ( Fig. 4a ) and (RMSD, SASA_np) ( Fig. 4b ). The tip4p/ ε model produces free-energy maps similar to those of tip4p/2005 ( Supplementary Fig. 3 ). The computed free-energy maps follow a typical two-state-like behaviour with a well-defined transition state. In comparison of the cold and heat denatured states on the free-energy representation, the former is substantially localized, whereas the latter state is broadly distributed over the RMSD space (See Fig. 4a ). As illustrated in Fig. 4 , at T max , the native state, which is located near (RMSD, N HB )=(1.0 Å, 7) or (RMSD, SASA_np)=(1.0 Å, 600.0 Å 2 ), is more populated than non-native states. On cooling from T max to T low , the cold-denatured state incrementally emerged as a major population at either (RMSD, N HB )=(2.5 Å, 0) ( Fig. 4a ) or (RMSD, SASA_np)=(2.5 Å, 660 Å 2 ) ( Fig. 4b ). 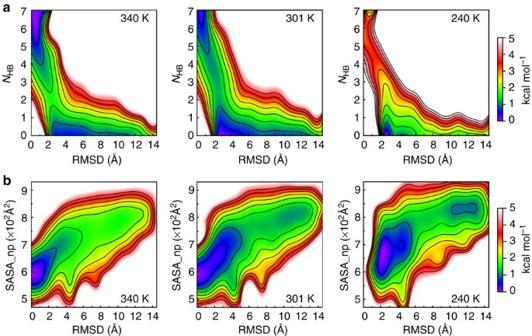Figure 4: Free-energy maps obtained using tip4p/2005. The conformational free-energy surfaces were shown at 240, 301 and 340 K. Two sets of reaction coordinates were employed for the free-energy representation: (a)NHBversus RMSD. (b) SASA_np versus RMSD. Figure 4: Free-energy maps obtained using tip4p/2005. The conformational free-energy surfaces were shown at 240, 301 and 340 K. Two sets of reaction coordinates were employed for the free-energy representation: ( a ) N HB versus RMSD. ( b ) SASA_np versus RMSD. Full size image In general, the strength of hydrophobic forces decreases on decreasing temperature [3] . During cold denaturation, this weakening hydrophobic force can disrupt the native hydrophobic cluster of the β-hairpin peptide. Thus, non-polar groups of MrH1, if exposed to water, will increase their SASA [26] . This behaviour is clearly illustrated in the free-energy surface of (RMSD, SASA_np) ( Fig. 4b ), where the non-polar component of SASA is shown to increase as the temperature decreases. Probing water ordering around hydrophobic residues Capturing detailed ordering pictures of water around hydrophobic residues is fundamentally important to elucidate the role of water in cold denaturation. In an attempt to seek a possibility of such water-ordering behaviours, tetrahedral order parameters of water [27] were computed at T low and T max . 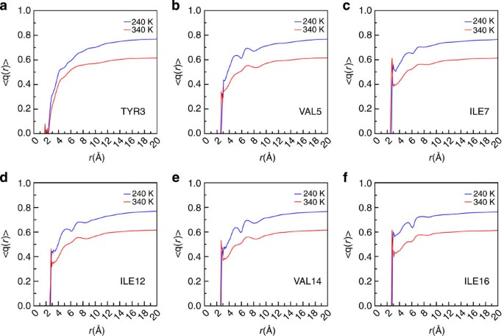Figure 5: Tetrahedral order parameters of water near non-polar residues. Using the tip4p/2005 water model, the tetrahedral order parameters of water at 240 and 340 K were calculated as a function of the radial distance from each centre of six hydrophobic residues of the β-hairpin peptide. The six hydrophobic residues are (a) TYR3, (b) VAL5, (c) ILE7, (d) ILE12, (e) VAL14 and (f) ILE16. Note that this order parameter is 1 for a perfect tetrahedral configuration. Figure 5 represents the radial-dependent tetrahedral order parameters of water around each of the six non-polar residues. This result indicates that the tetrahedral order of water increases with decreasing temperature, but the water ordering near non-polar residues is not pronounced and even less than that of bulky water (see also the water/non-polar residue pair distribution functions in Supplementary Fig. 4 ). Hence, the lack of tetrahedral ordering of the interfacial water would prevent the formation of optimal hydrogen bonds during cold denaturation. Therefore, in contrast with the previously suggested iceberg-like structure model [2] , the enthalpic compensation of the entropy loss via enhanced water ordering around hydrophobic residues could not be a driving force for the cold denaturation of MrH1, suggesting that the system entropy loss must come from other sources of water. In an effort to gain more insights into cold denaturation, we decomposed the system enthalpy change into several contributing terms and also calculated the change of SASA on unfolding (Δ SASA F → D ) ( Table 2 ). For all three water models, as the MrH1 unfolds, its Δ SASA F → D increases, thereby increasing water-excluded volume. Thus, regardless of the nature of explicit water models, it is expected that protein unfolding accompanies a substantial loss of the translational water entropy due to such increased water-excluded volume effects. Furthermore, Δ SASA F → D is an increasing function of temperature and its temperature-dependent behaviour is different for each water model. On cooling from T max to T low , Δ SASA F → D decreases much less for the tip3p than the tip4p models, so that the alleviation of translational entropy loss of the tip3p water is not sufficient enough to stabilize the unfold state at T low . Hence, for the tip3p water, the temperature should be lowered further below T low to observe the cold-denatured state in the major population. For the modified tip4p models; however, the positive contribution of Δ SASA F → D on the cold denaturation at T low is much smaller than that on the unfolding at T max ( Table 2 ). Therefore, this reduction of the translational entropy of the tip4p water becomes less severe at T low, thereby effectively decreasing the hydration free-energy cost of the unfold state for cold denaturation. Consistent with previous studies [28] , [29] , [30] , [31] , this temperature-dependent behaviour of the translational water entropy seems to be a plausible interpretation of the cold-denaturation phenomenon of MrH1. Figure 5: Tetrahedral order parameters of water near non-polar residues. Using the tip4p/2005 water model, the tetrahedral order parameters of water at 240 and 340 K were calculated as a function of the radial distance from each centre of six hydrophobic residues of the β-hairpin peptide. The six hydrophobic residues are ( a ) TYR3, ( b ) VAL5, ( c ) ILE7, ( d ) ILE12, ( e ) VAL14 and ( f ) ILE16. Note that this order parameter is 1 for a perfect tetrahedral configuration. Full size image Table 2 Various terms on changing from the fold to denatured state. Full size table As summarized in Table 2 , on unfolding, the enthalpic contributions from protein ( ) and water ( ) are increasing functions of temperature, whereas the contribution from protein/water intermolecular interactions ( ) is a decreasing function of temperature. Therefore, only and terms can be responsible for decreasing the system enthalpy on cold denaturation. It is of interest to note that the temperature dependence of , which is the water reorganization energy on unfolding, appears to contribute more to the loss of system enthalpy on unfolding at low temperatures. Refolding dynamics initiating from cold-denatured state As the complete pictures of free-energy landscapes were obtained during cooling, we decided to probe the dynamics of refolding at T max . At this temperature, the cold-denatured-like state is placed in the non-native basin of the free-energy surface ( Fig. 4a ). Starting from this state, several refolding MD simulations at T max =340 K and P =1 atm were attempted using tip4p/2005. Two successful examples of fast refolding trajectories are shown in Fig. 6 , where the values of RMSD, N HB and SASA_np are traced in time. These refolding events, which occur in only several hundred nano-seconds, indicate that the β-turn (type I’) is formed first and followed by a concurrent formation of the hydrophobic core packing and the native hydrogen bond. 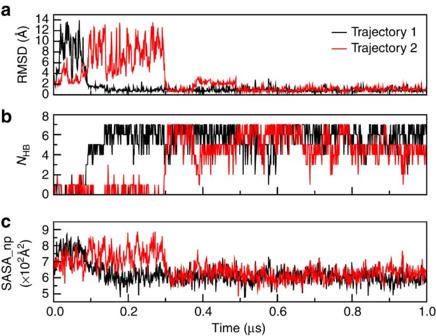Figure 6: Refolding MD trajectories starting from the cold-denatured-like state. Two successful refolding trajectories atTmax=340 K using tip4p/2005 are shown for 1 μs. The first refolding event to the native state occurs in 200 ns and 320 ns for trajectories 1 and 2, respectively. The refolding trajectories are shown with (a) RMSD versus time, (b)NHBversus time and (c) SASA_np versus time. Figure 6: Refolding MD trajectories starting from the cold-denatured-like state. Two successful refolding trajectories at T max =340 K using tip4p/2005 are shown for 1 μs. The first refolding event to the native state occurs in 200 ns and 320 ns for trajectories 1 and 2, respectively. The refolding trajectories are shown with ( a ) RMSD versus time, ( b ) N HB versus time and ( c ) SASA_np versus time. Full size image A state-of-the-art REMD simulation at all-atom levels under constant pressure enables us to observe the cold-denaturation-like process of a β-hairpin peptide (MrH1) and to characterize a possible candidate of cold-denatured structures at low temperatures. Direct comparisons of the simulation results based on three different water models indicate that improved modelling of temperature dependence of water is one contributing factor for cold denaturation as shown by the case of two improved tip4p models, but may not be a necessary condition as shown by the case of the tip3p model. According to the multiple snapshots of free-energy landscapes on cooling, at ambient temperatures the native state of MrH1 is slightly more populated than the non-native state. On decreasing temperature, however, the cold-denatured sate population grows and eventually this state becomes the lowest free-energy minimum at low temperatures. The most plausible conformation of the cold-denatured state of MrH1 retains relatively a compact backbone structure somewhat close to that of the native state, but exhibits a significant loss of native hydrogen bonds, a disruption of type I′-turn, and water-exposed hydrophobic residues. In the minor conformations of this state, more disruption of the native β-strand is observed. All these major and minor conformations relevant to this cold-denatured-like state exhibit a common structural feature of collapsed states. Owing to the marginal stability of the fold state and the small size of MrH1, this model peptide may display substantial conformational diversity and fluctuation in the fold-state ensemble, thereby making a different interpretation on the cold-denatured state possible. Presumably, the cold-denatured state that we have identified could be another fold state without native backbone hydrogen bonds and hydrophobic clustering. Therefore, a possibility that an alternative low-lying free-energy state is being captured at low temperatures may not be completely ruled out. In contrast with the previously proposed iceberg-like model [2] , the current simulation result showed that interfacial water in the vicinity of non-polar residues is apparently less ordered than the bulk water. Therefore, the lack of such orientational ordering of water at low temperatures precludes a possibility of enhanced water hydrogen-bond networks near hydrophobic residues. Instead, as proposed in earlier studies [28] , [29] , [30] , [31] , the entropy loss on cold denaturation is more likely attributed to the effect of translational entropy of water coexisting with proteins. Native state modelling The coordinates of the NMR native structure of the β-hairpin peptide (MrH1) are not directly available from the literatures. Hence, the native structure of this peptide was computer-modeled by taking advantage of 30 NMR φ / ψ angle restraint data [12] . This peptide is then solvated by a total of 2,577 water molecules ions in a dodecahedron box of a size 48.4 Å. For charge neutralization, 4 Cl − were added to the system. Using the ff99sb-nmr1-ildn force field in combination with the tip3p model, the whole system is minimized with the steepest-decent method and then equilibrated for 500 ns using an isothermal–isobaric MD ( T =300 K and P =1.0 atm). The final structure was taken to be the native NMR structure ( Supplementary Fig. 1a,b ) and used as a reference to compute the RMSD value of peptide conformations. This native NMR model fully satisfied the NMR torsional angle restraint result ( Supplementary Fig. 1c,d ). Simulation details For all MD simulations, a time step of 4 fs was chosen using the virtual interaction site scheme by Feenstra et al. [32] The modified Berendsen thermostat [33] and the Parrinello–Rahman barostat [34] were employed to control system temperature and pressure, respectively. The cutoff distance for non-bond interactions including van der Waals and coulomb interactions (particle mesh Ewald) was set to 10 Å. In the in silico cold-denaturation study, a REMD method was used in the NPT ensemble [35] . A total of 70 replicas were assigned to cover the temperature range 240–498.9 K. Initially, these replica temperatures were generated by using the scheme of Patriksson and Spoel [36] and a preliminary REMD simulation was carried out for 100 ns. On the basis of this simulation, replica temperatures were readjusted for better overlaps of energy distributions between adjacent temperatures. For all replicas, setting all replica pressures to 1 atm caused numerical instability resulting from exchanging high-temperature replicas above 100 °C owing to their large volume fluctuations. To circumvent this problem, for temperatures below 100 °C, the system pressure was set to 1 atm as usual, but at above 100 °C, it was assigned in exponentially increasing order to maintain the density of system at that of the replica near 100 °C ( Supplementary Fig. 5a,b ). Average system density for each choice of water models was plotted versus all replica temperatures ( Supplementary Fig. 5c ). The replica exchange in REMD was attempted every 4 ps and the acceptance ratio of exchange events is 19−40% ( Supplementary Fig. 5d ). For the tip3p and the tip4p/2005, REMD simulation, initiating from the native state, was run for 2 μs for each replica (a total of 140 μs). In the case of tip4p/ ε , noting that the tip4p/ ε model behaves in the same manner as tip4p/2005, the preequilibrated ensemble obtained with tip4p/2005 was utilized as an initial condition for the REMD run using tip4p/ ε . In this case, a simulation length of 1 μs per replica (a total of 70 μs) appeared to be sufficient. In an effort to show the convergence of the current REMD simulation, the number of folded replicas is monitored in time. The time profile of number of folded replicas in the REMD initiating from the native state reached a steady state in 700 ns for both tip3p and tip4p/2005 and in 200 ns for tip4p/ ε ( Supplementary Fig. 6a ). As a result, such non-equilibrium trajectories in the initial periods of 700 ns and 200 ns were discarded to calculate ensemble averages. As a further convergence test on the present REMD simulation, another round of REMD simulations was performed for 1.5 μs per replica starting from the cold-denatured state. This additional simulation result clearly showed that the number of folded replicas in time approached the steady-state value of the simulation starting from the native state ( Supplementary Fig. 6b ). The free-energy map was computed using where P ( X, Y ) is the equilibrium probability of finding protein conformations at reaction coordinates X and Y , R is the gas constant and T is the absolute temperature. To compute the melting curves (folding fraction versus temperature), the folding state was defined if N HB ≥2.5. This criterion well distinguishes the native basin from the non-native one on the free-energy surface of (RMSD, N HB ) at T max . In this work, the RMSD criterion is also a possible choice, but somewhat difficult to distinguish fold states from unfold states, as the RMSD distributions of the native and the cold-denatured states tend to overlap with each other (See Fig. 4a ). Nevertheless, one can still use the RMSD criterion by employing Gaussian curve decomposition in RMSD space to circumvent such overlapping problem in the RMSD space. It is of note that the folding fraction obtained from this Gaussian curve decomposition agrees well with one obtained from the criterion of N HB ≥2.5. All simulations and analyses were performed using the GROMACS programme [37] . Thermodynamic parameters from two-state folding model Assuming two-state folding and temperature-independent heat capacity, the folding fraction f is given by [12] where Δ H °, Δ S ° and Δ C ° P are the changes of enthalpy, entropy and heat capacity on unfolding, respectively. The equations (2, 3, 4) were used to determine Δ H ° 298 K , Δ S ° 298 K and Δ C ° P by curve fit to the simulated melting curves ( f versus T ). Tetrahedral order parameter The local tetrahedral order parameter [38] is defined as where ψ ikj is the angle formed by the three water oxygen atoms of the centre water molecule k and its nearest neighbour water molecules i and j . On the basis of this definition, the tetrahedral order parameter of water molecules at a distance r from a reference point [27] is calculated by using where n ( r , Δ r ) is all the water molecules that are located at ( r , r +Δ r ) and r k is the position of water molecule k . The position of a water molecule is calculated using that of the oxygen atom (OW). How to cite this article: Yang, C. et al. A fully atomistic computer simulation study of cold denaturation of a β-hairpin. Nat. Commun. 5:5773 doi: 10.1038/ncomms6773 (2014).